PKA-induced dimerization of the RhoGAP DLC1 promotes its inhibition of tumorigenesis and metastasis Deleted in Liver Cancer 1 (DLC1) is a tumour suppressor that encodes a RhoGTPase-activating protein (RhoGAP) and is frequently inactivated in many human cancers. The RhoGAP activity of DLC1 against Rho signalling is well documented and is strongly associated with the tumour suppressor functions of DLC1. However, the mechanism by which the RhoGAP activity of DLC1 is regulated remains obscure. Here, we report that phosphorylation of DLC1 at Ser549 by cyclic AMP-dependent protein kinase A contributes to enhanced RhoGAP activity and promotes the activation of DLC1, which suppresses hepatoma cell growth, motility and metastasis in both in vitro and in vivo models. Intriguingly, we found that Ser549 phosphorylation induces the dimerization of DLC1 and that inducible dimerization of DLC1 can rescue the tumour suppressive and RhoGAP activities of DLC1 containing a Ser549 deletion. Our study establishes a novel regulatory mechanism for DLC1 RhoGAP activity via dimerization induced by protein kinase A signalling. Deleted in Liver Cancer (DLC) family members are tumour suppressors with a high degree of structural similarity [1] , [2] , [3] . Compelling evidence has shown that DLC members are frequently inactivated in many human cancers [4] , and studies have demonstrated their inhibitory roles in tumorigenesis, angiogenesis and metastasis in various cancer models [5] , [6] , [7] , [8] . DLC1 was the first identified member of the DLC family and is the best characterized [3] . DLC1 localizes to focal adhesions and functions as a Rho GTPase-activating protein (RhoGAP), which negatively regulates RhoA, RhoB, RhoC and CDC42 proteins [9] . Rho proteins are important regulators of normal biological processes, such as actin cytoskeleton organization, transcription, cell motility and cell proliferation. However, the activation of Rho proteins contributes to tumorigenesis and metastasis in many cancers [10] , and RhoGAP activity has a predominant role in the tumour suppressor functions of DLC1 [11] . In different cell line models, ectopic expression of the RhoGAP mutant of DLC1 fails to suppress cell growth and motility [12] , [13] , and functional studies have shown that RhoGAP and the growth inhibitory activities of DLC1 are impaired as a result of T301K and S308I mutations, which were identified in prostate and colon cancer patients [14] . These studies suggest that RhoGAP activity and growth suppression activity are tightly associated. In a mouse model, knockdown of DLC1 was shown to cooperate with Myc to promote hepatocarcinogenesis [8] . In addition, mouse hepatoma cells with silenced DLC1 exhibit increased active RhoA levels and actin stress fibre formation, which provides overwhelming evidence for the activation of Rho as a consequence of deregulated DLC1 and stresses the importance of DLC1 RhoGAP activity in tumorigenesis in vivo . Nevertheless, RhoGAP-independent signalling may also contribute to the biological activities of DLC1 in different cellular contexts [6] , [7] , [15] , [16] , [17] . Therefore, it is important to comprehend how the RhoGAP activity of DLC1 is regulated and associated with its functional effects in cancer cells. It has been reported that Ras-GAP interacts with DLC1 at focal adhesions [18] . In addition, the overexpression of Ras-GAP was shown to impair the growth inhibitory activity of DLC1 and increase the RhoA level in cells, suggesting that Ras-GAP is a negative regulator of the RhoGAP activity of DLC1. Additionally, the association of DLC1 and phosphatidylinositol-4,5-bisphosphate (PI(4,5)P 2 ) is known to stimulate RhoGAP activity [19] , and interaction-defective DLC1 is less efficient at suppressing Rho and inhibiting cell migration and proliferation. Recent studies have also demonstrated that phosphorylation is an additional regulatory mechanism for DLC1 activation, whereby activated protein kinase C (PKC) and protein kinase D (PKD) phosphorylate DLC1 and promote the association of DLC1 and 14-3-3 adaptor protein, leading to the blockade of RhoGAP activity [20] . The RhoGAP domain was also shown to be directly phosphorylated by PKD at Ser807, although the in vitro RhoGAP activity remained unaffected [21] . In this study, we focused on how PKA phosphorylates and governs the biological functions of DLC1 in vitro and in vivo . Our findings reveal a novel mechanism by which PKA-induced dimerization of DLC1 results in the enhanced RhoGAP and inhibitory activities of DLC1. PKA phosphorylates DLC1 at Ser431 and Ser549 An in silico analysis of the DLC1 protein sequence revealed two consensus phospho-PKA substrate (pPKAS) motifs at amino acids 428–431 (RRNS*) and 546-549 (RRDS*) ( Fig. 1a ). Thus, we evaluated whether PKA phosphorylates DLC1. An anti-pPKAS antibody that specifically recognizes the phosphorylated PKAS motif was used to detect the phosphorylation of DLC1 following the activation of PKA signalling. When Myc-DLC1 was coexpressed with the PKA catalytic subunit (PKA-Cα) in HEK293T cells, phosphorylation of immunoprecipitated Myc-DLC1 was detected ( Fig. 1b ). Moreover, the phosphorylation of DLC1 was enhanced by forskolin treatment, a known activator of PKA, and phosphorylation of DLC1 was suppressed in the presence of H-89, an inhibitor of PKA ( Fig. 1c ). The association between DLC1 and PKA-Cα was then revealed by co-immunoprecipitation ( Fig. 1d ), and an in vitro kinase assay demonstrated that recombinant PKA-Cα could directly phosphorylate the GST-DLC1 349-645 fusion protein ( Fig. 1e ). Furthermore, forskolin stimulation induced the phosphorylation of endogenous DLC1 in HLE cells ( Fig. 1f ). 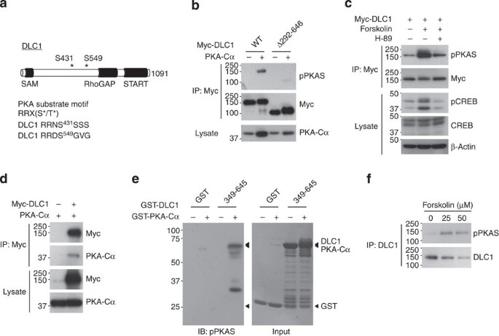Figure 1: DLC1 is a substrate of PKA. (a) Schematic diagram of the DLC1 protein showing two consensus PKA substrate motifs, RRX(S*/T*), in the central region of DLC1. R, arginine; S* and T*, phosphorylated serine and threonine; X, any amino acid. (b) Phosphorylated residue(s) located in the central region of DLC1. DLC1 and the Δ292-646 mutant expressed with or without PKA-Cα in HEK293T cells were immunoprecipitated using an anti-Myc antibody and detected with an anti-pPKAS antibody. (c) Phosphorylation of DLC1 is enhanced following forskolin treatment and is suppressed by the addition of the H-89 inhibitor in HEK293T cells. (d) Myc-DLC1 and PKA-Cα interact in cells. HEK293T cell lysates transfected with Myc-DLC1 and PKA-Cα were immunoprecipitated with an anti-Myc antibody and then immunodetected with the anti-PKA-Cα antibody. (e) PKA-Cα directly phosphorylates DLC1in vitro. Anin vitrokinase assay demonstrating the purified GST-DLC1 fusion protein (349-645) incubated with or without recombinant PKA-Cα. (f) Phosphorylation of endogenous DLC1 in HLE cells is enhanced by forskolin stimulation. Figure 1: DLC1 is a substrate of PKA. ( a ) Schematic diagram of the DLC1 protein showing two consensus PKA substrate motifs, RRX(S*/T*), in the central region of DLC1. R, arginine; S* and T*, phosphorylated serine and threonine; X, any amino acid. ( b ) Phosphorylated residue(s) located in the central region of DLC1. DLC1 and the Δ292-646 mutant expressed with or without PKA-Cα in HEK293T cells were immunoprecipitated using an anti-Myc antibody and detected with an anti-pPKAS antibody. ( c ) Phosphorylation of DLC1 is enhanced following forskolin treatment and is suppressed by the addition of the H-89 inhibitor in HEK293T cells. ( d ) Myc-DLC1 and PKA-Cα interact in cells. HEK293T cell lysates transfected with Myc-DLC1 and PKA-Cα were immunoprecipitated with an anti-Myc antibody and then immunodetected with the anti-PKA-Cα antibody. ( e ) PKA-Cα directly phosphorylates DLC1 in vitro . An in vitro kinase assay demonstrating the purified GST-DLC1 fusion protein (349-645) incubated with or without recombinant PKA-Cα. ( f ) Phosphorylation of endogenous DLC1 in HLE cells is enhanced by forskolin stimulation. Full size image To determine whether Ser431 and Ser549 of DLC1 are targets of PKA, we created and analysed the phosphorylation of an internal deletion mutant of DLC1, Δ292-646 ( Fig. 2a ). When the deletion mutant was coexpressed with PKA-Cα in HEK293T cells, no phosphorylation was detected in the Δ292-646 mutant ( Fig. 1b ). We then validated the identity of the phosphorylated residue(s) by creating phospho-defective mutants (S431A, S549A and S431AS549A) and generating phospho-DLC1 (pDLC1) antibodies that specifically recognize pSer431 and pSer549. Under forskolin stimulation or coexpression with PKA-Cα, DLC1 was phosphorylated at Ser431 and Ser549 in HEK293T cells, whereas this phosphorylation was lost in the S431A and S549A mutants, as detected using the anti-pDLC1 (Ser431) and anti-pDLC1 (Ser549) antibodies, respectively ( Fig. 2b and Supplementary Fig. S1 ). Additionally, S431 phosphorylation was largely reduced in the S549A mutant as compared with wild-type (WT) DLC1 following forskolin stimulation. Conversely, Ser431 was robustly phosphorylated in the S549D phosphomimetic mutant even without forskolin stimulation, which suggests that Ser431 phosphorylation is dependent on the phosphorylation status of Ser549. To determine the effect of PKA on the phosphorylation of DLC1 at Ser431 and Ser549, PKA-Cα expression was suppressed in HEK293T cells. As shown in Fig. 2c , forskolin-induced phosphorylation at Ser431 and Ser549 was largely reduced in PKA-Cα knockdown cells. In addition, the phosphorylation of endogenous DLC1 at Ser431 and Ser549 in HLE cells following forskolin stimulation was demonstrated using anti-pDLC1 antibodies ( Fig. 2d ). Direct phosphorylation of DLC1 by PKA was further validated using the in vitro kinase assay with recombinant DLC1 mutants and PKA-Cα ( Fig. 2e ). 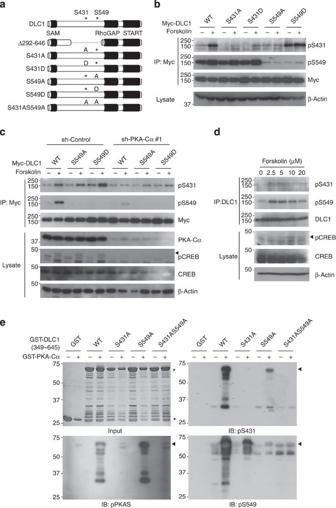Figure 2: PKA phosphorylates DLC1 at Ser341 and Ser549. (a) Schematic representation of DLC1 and its mutants used in the study. Two consensus PKA substrate motifs are shown, and Ser431 and Ser549 are the potential phosphorylated residues. An internal deletion mutant, a phospho-defective (SA) mutant and a phosphomimetic mutant (SD) of DLC1 were created. (b) Ser431 phosphorylation is dependent on the phosphorylation of Ser549. The phospho-defective and phosphomimetic mutants of DLC1 were subjected to immunoprecipitation and immunodetection. (c) Knockdown of PKA-Cα suppresses the phosphorylation of DLC1. The phosphorylation of Myc-DLC1, -S549A and -S549D was examined and compared in stable sh-PKA-Cα knockdown and sh-control clones. (d) Phosphorylation at Ser431 and Ser549 of endogenous DLC1. Endogenous DLC1 in HLE cells following forskolin stimulation was immunoprecipitated using an anti-DLC1 antibody followed by immunoblotting using anti-pS431 and -pS549 antibodies. (e) PKA-Cα phosphorylates DLC1 at Ser431 and Ser549in vitro. Thein vitrokinase assay was performed using purified GST-DLC1, GST-S431A, GST-S549A and GST-S431AS549A fusion proteins incubated with or without recombinant GST-PKA-Cα in the presence of ATP. Phosphorylation was detected using anti-pPKAS, -pS431 and -pS549 antibodies. The asterisk indicates the input of GST-DLC1 and GST- PKA-Cα. The arrowhead denotes the phosphorylation of DLC1. Figure 2: PKA phosphorylates DLC1 at Ser341 and Ser549. ( a ) Schematic representation of DLC1 and its mutants used in the study. Two consensus PKA substrate motifs are shown, and Ser431 and Ser549 are the potential phosphorylated residues. An internal deletion mutant, a phospho-defective (SA) mutant and a phosphomimetic mutant (SD) of DLC1 were created. ( b ) Ser431 phosphorylation is dependent on the phosphorylation of Ser549. The phospho-defective and phosphomimetic mutants of DLC1 were subjected to immunoprecipitation and immunodetection. ( c ) Knockdown of PKA-Cα suppresses the phosphorylation of DLC1. The phosphorylation of Myc-DLC1, -S549A and -S549D was examined and compared in stable sh-PKA-Cα knockdown and sh-control clones. ( d ) Phosphorylation at Ser431 and Ser549 of endogenous DLC1. Endogenous DLC1 in HLE cells following forskolin stimulation was immunoprecipitated using an anti-DLC1 antibody followed by immunoblotting using anti-pS431 and -pS549 antibodies. ( e ) PKA-Cα phosphorylates DLC1 at Ser431 and Ser549 in vitro . The in vitro kinase assay was performed using purified GST-DLC1, GST-S431A, GST-S549A and GST-S431AS549A fusion proteins incubated with or without recombinant GST-PKA-Cα in the presence of ATP. Phosphorylation was detected using anti-pPKAS, -pS431 and -pS549 antibodies. The asterisk indicates the input of GST-DLC1 and GST- PKA-Cα. The arrowhead denotes the phosphorylation of DLC1. Full size image Ser549 is conserved among the DLC family Members of the DLC family share high sequence homology and structural similarity [1] . Based on the sequence alignment, Ser549 was found to be conserved among DLC1, DLC2 and DLC3 ( Supplementary Fig. S2a ). Ser549 of DLC1 corresponds to Ser572 and Ser561 of DLC2 and DLC3, respectively. The anti-pPKAS antibody detected the phosphorylation of immunoprecipitated GFP-DLC2 when PKA-Cα was coexpressed in HEK293T cells ( Supplementary Fig. S2b ). Because PKAS motifs are conserved within the family, we used the anti-pS549 antibody to detect DLC2 phosphorylation following forskolin stimulation. The anti-pPKAS and anti-pS549 antibodies were both able to detect the enhanced phosphorylation of immunoprecipitated FLAG-DLC2 ( Supplementary Fig. S2c ). However, phosphorylation was completely abolished in the S572A phospho-defective mutant of DLC2 following forskolin stimulation, suggesting that Ser572 of DLC2 is indeed a target of PKA ( Supplementary Fig. S2d ). Ser549 phosphorylation regulates DLC1 biological activities We then conducted a colony formation assay to address the functional differences between DLC1 and its phospho-defective and phosphomimetic mutants of Ser431 and Ser549. WT DLC1 and the mutants were assessed based on their ability to suppress SMMC7721 cell growth ( Supplementary Fig. S3a ), and we found that the S431A and S431D mutants displayed similar inhibitory activity as compared with WT DLC1, suggesting that the phosphorylation status of Ser431 alone did not mediate the biological activity of DLC1. Intriguingly, the S549A mutant failed to inhibit colony formation, whereas the S549D mutant enhanced the inhibitory effect of colony formation. To corroborate the physiological relevance of DLC1 Ser549 phosphorylation, we used a luciferase-labelled mouse p53 null hepatoblast cell line expressing an oncogenic Ras, which has previously been used to characterize the functions of DLC1 [6] , [8] . Stable clones of DLC1 WT, S549A and S549D were established in mouse hepatoma cells ( Fig. 3a and Supplementary Fig. S3b ), and the results demonstrated that the S549A mutant lost its inhibitory activity, whereas the S549D mutant enhanced the suppression of proliferation and led to anchorage-independent growth of the hepatoma cells ( Fig. 3b ). Furthermore, flow cytometry analysis revealed that the S549D stable clone had a remarkable sub-G1 population of cells ( Fig. 3d ). In the in vivo model, the expression of WT DLC1 and the S549D mutant efficiently suppressed the tumour development of subcutaneously injected hepatoma cells ( Fig. 3e ) and resulted in tumours with a smaller size as compared with the vector control and S549A-expressing tumours ( n =8) ( Fig. 3f ). The loss of inhibitory activity in the S549A mutant indicated the dependence of Ser549 phosphorylation for DLC1 function. 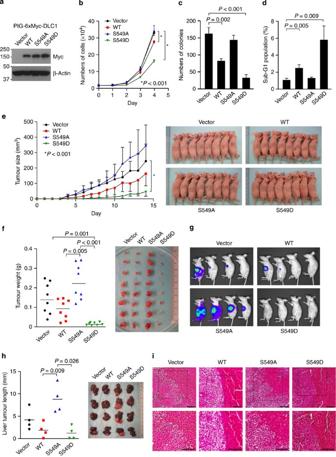Figure 3: Phosphorylation at Ser549 enhances the growth suppression activity of DLC1. (a) Western blot analysis confirming the stable expression of DLC1 and its mutants in mouse hepatoma cells. (b) Expression of DLC1 WT and S549D inhibits cell proliferation. Growth curves of mouse hepatoma clones stably expressing WT, S549A, S549D and a control clone were measured. (n=3 for each group) (c) Expression of DLC1 WT and S549D suppresses anchorage-independent growth. Stable clones of DLC1 were studied in a soft agar assay, and colonies were imaged and counted after 3 weeks of incubation (n=3 for each group). (d) Ser549 phosphorylation enhances the apoptosis-inducing activity of DLC1. The DNA content of DLC1 stable clones was determined by flow cytometry. The percentage of the sub-G1 population was determined (n=3 for each group). (e) Expression of DLC1 WT and S549D inhibitsin vivotumorigenicity. DLC1 stable clones were inoculated into nude mice, and tumour size was measured during the course of the experiment (n=8 for each group). (f) DLC1 and S549D suppress tumour development. Tumours were excised and weighed at the end of the experiments. (g) Expression of S549A promotes tumour formation in the mouse liver. Orthotopic liver implantation of hepatoma cells stably expressing DLC1 was performed. Animals were examined by bioluminescence at 3 weeks after implantation (n=4 for each group). (h) Expression of S549D results in the smallest tumours in the mouse liver. Livers were resected, and the size of tumours was measured. (i) Tumours derived from WT and S549D stable cells display less aggressive growth fronts than the vector and S549A stable cells. H&E staining of liver tissues from mice implanted with xenografts derived from DLC1 stable clones. An enlarged view of the tumour growth in front of the implanted xenografts is shown below. Scale bar, 100 μm. Error bar represents s.d. The results are expressed as the mean±s.d. *P<0.001. Figure 3: Phosphorylation at Ser549 enhances the growth suppression activity of DLC1. ( a ) Western blot analysis confirming the stable expression of DLC1 and its mutants in mouse hepatoma cells. ( b ) Expression of DLC1 WT and S549D inhibits cell proliferation. Growth curves of mouse hepatoma clones stably expressing WT, S549A, S549D and a control clone were measured. ( n =3 for each group) ( c ) Expression of DLC1 WT and S549D suppresses anchorage-independent growth. Stable clones of DLC1 were studied in a soft agar assay, and colonies were imaged and counted after 3 weeks of incubation ( n =3 for each group). ( d ) Ser549 phosphorylation enhances the apoptosis-inducing activity of DLC1. The DNA content of DLC1 stable clones was determined by flow cytometry. The percentage of the sub-G1 population was determined ( n =3 for each group). ( e ) Expression of DLC1 WT and S549D inhibits in vivo tumorigenicity. DLC1 stable clones were inoculated into nude mice, and tumour size was measured during the course of the experiment ( n =8 for each group). ( f ) DLC1 and S549D suppress tumour development. Tumours were excised and weighed at the end of the experiments. ( g ) Expression of S549A promotes tumour formation in the mouse liver. Orthotopic liver implantation of hepatoma cells stably expressing DLC1 was performed. Animals were examined by bioluminescence at 3 weeks after implantation ( n =4 for each group). ( h ) Expression of S549D results in the smallest tumours in the mouse liver. Livers were resected, and the size of tumours was measured. ( i ) Tumours derived from WT and S549D stable cells display less aggressive growth fronts than the vector and S549A stable cells. H&E staining of liver tissues from mice implanted with xenografts derived from DLC1 stable clones. An enlarged view of the tumour growth in front of the implanted xenografts is shown below. Scale bar, 100 μm. Error bar represents s.d. The results are expressed as the mean±s.d. * P <0.001. Full size image We also performed orthotopic liver implantation using tumours derived from the mouse hepatoma stable clones. Three weeks after liver implantation, Xenogen imaging revealed inhibition of tumour growth in the livers of mice with DLC1 WT and S549D tumours, whereas accelerated tumour growth was observed in mice with S549A tumours ( n =4) ( Fig. 3g ). DLC1- and S549D-implanted tumours were smaller in size, and the largest tumours were found in mice implanted with S549A cells as compared with control animals ( Fig. 3h ). Histological analysis revealed that DLC1 and S549D tumours exhibited an expansile growth front, whereas both the vector control and S549A tumours had more irregular growth fronts ( Fig. 3i ). Tumour microsatellite formation was also observed in the S549A group ( Supplementary Fig. S3c ). Xenogen imaging of excised lungs further revealed the most prominent metastasis in the S549A group ( Supplementary Fig. S3d,e,f ). DLC1 has been shown to act as a metastasis suppressor in different cancer models [5] , [6] , [22] . DLC1 impeded the migratory ability and invasiveness of hepatoma cells, as indicated by the decrease in the numbers of migrated and invaded cells, respectively ( Fig. 4a ). However, expression of S549A had no suppressive effect on either the migration or invasion of the cells. In contrast, S549D largely reduced the numbers of migrated and invaded cells in both assays. An experimental metastasis model using an intravenous injection of hepatoma cells revealed that all mice ( n =4) injected with the control and S549A cells had remarkable lung metastasis. Conversely, less prominent lung metastases were observed in all mice injected with DLC1 and minor metastasis was only observed in 2 of 4 mice injected with S549D cells ( Fig. 4c ). In accordance with the size of the lung metastases, mice injected with the vector control or S549A died within 3 weeks of the injection, whereas mice injected with DLC1 cells survived for 25 days. Mice injected with S549D cells had the longest survival among all groups and were killed on day 25 ( Fig. 4d ). Histological analysis of the excised lungs revealed large and prominent tumour foci in the control and S549A groups, whereas smaller tumour foci were observed in the DLC1 group ( Fig. 4e ). Furthermore, a dramatic reduction in distant metastases was observed in the S549D group. Collectively, these results demonstrate that S549 phosphorylation stimulates the growth and metastasis inhibitory activities of DLC1. 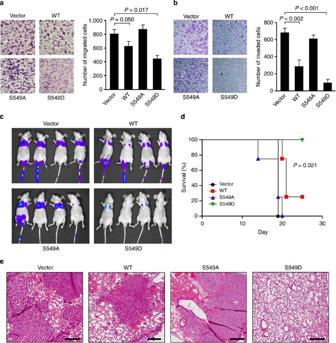Figure 4: Metastasis inhibitory activity of DLC1 is promoted by Ser549 phosphorylation. (a) Ser549 phosphorylation enhances the inhibitory activity of DLC1 with respect to cell migration. Migration of DLC1 stable clones was assessed using a Transwell assay (n=3 for each group). (b) Ser549 phosphorylation enhances the inhibitory activity of DLC1 with respect to cell invasion. The invasiveness of DLC1 stable clones was determined using a Matrigel-coated invasion chamber (n=3 for each group). (c) Lung metastasis evaluated according to the luciferase signal at 3 weeks post intravenous injection of hepatoma cells into mice (n=4 for each group). (d) Survival curve of mice subjected to tail vein injection of hepatoma cells. Mice from the S549D group were sacrificed on day 25. (e) Representative images of H&E-stained lung tissue. Lungs were excised and examined for tumour focus formation by histological analysis. Scale bar, 100 μm. Error bar represents s.d. The results are expressed as the mean±s.d. Figure 4: Metastasis inhibitory activity of DLC1 is promoted by Ser549 phosphorylation. ( a ) Ser549 phosphorylation enhances the inhibitory activity of DLC1 with respect to cell migration. Migration of DLC1 stable clones was assessed using a Transwell assay ( n =3 for each group). ( b ) Ser549 phosphorylation enhances the inhibitory activity of DLC1 with respect to cell invasion. The invasiveness of DLC1 stable clones was determined using a Matrigel-coated invasion chamber ( n =3 for each group). ( c ) Lung metastasis evaluated according to the luciferase signal at 3 weeks post intravenous injection of hepatoma cells into mice ( n =4 for each group). ( d ) Survival curve of mice subjected to tail vein injection of hepatoma cells. Mice from the S549D group were sacrificed on day 25. ( e ) Representative images of H&E-stained lung tissue. Lungs were excised and examined for tumour focus formation by histological analysis. Scale bar, 100 μm. Error bar represents s.d. The results are expressed as the mean±s.d. Full size image Ser549 phosphorylation induces the dimerization of DLC1 To understand the molecular basis for the PKA-modulated DLC1 effects, we investigated whether phosphorylation of Ser549 regulates the subcellular localization and interaction potentials of DLC1. The focal adhesion localization of DLC1 remained intact following forskolin treatment and was conserved for both the S549A and S549D mutants ( Supplementary Figs S4 and 5 ). DLC is a nucleocytoplasmic shuttling protein [20] , [23] , although this shuttling function was not affected by Ser549 phosphorylation. DLC1 interaction with tensin has been well established and is crucial for proper function of DLC1 [12] , [24] , [25] , [26] . Thus, we investigated whether Ser549 phosphorylation regulates the association between DLC1 and tensins. The results indicated that S549D and tensin2 had the strongest binding as compared with the binding of DLC1 and S549A to tensin2 ( Supplementary Fig. S6 ). Phosphorylation of Ser549 was also found to enhance the dimerization of DLC1. Myc-DLC1 weakly dimerized and displayed an enhanced interaction with FLAG-S549D but failed to interact with S549A in HEK293 cells ( Fig. 5a ). In addition, dimerization of DLC1 was enhanced with increasing durations of forskolin treatment ( Fig. 5b ). Phorbol-12,13-dibutyrate (PDBu), an analogue of diacylglycerol that has been shown to stimulate DLC1 phosphorylation at Ser327 and Ser431 and promote DLC1 association with 14-3-3 proteins [20] , was tested for its effect on DLC1 dimerization. Treatment of cells with PDBu-induced phosphorylation of Ser431 but not Ser549 and slightly promoted the dimerization of DLC1 ( Fig. 5c ). Further analysis of the interaction between the S549D mutant and various truncated mutants of DLC1 indicated that amino acids 500–685 of DLC1 were sufficient to mediate the dimerization of DLC1 ( Fig. 5d ). Using the GST-DLC 349-645 protein in a kinase assay, we found that GST-DLC1 349-645 dimerized in the presence of GST-PKA-Cα. The DLC1 dimer had a molecular size that was approximately twice that of the monomer, and the dimer formed in buffer without a reducing agent ( Fig. 5f ). These results indicate that the dimerization of DLC1 is dependent on PKA-mediated Ser549 phosphorylation. The conservation of Ser549 among DLC family members suggests that phosphorylation at the corresponding Ser572 in DLC2 may induce the dimerization of DLC2. Furthermore, DLC2 did not interact with the S572A phospho-defective mutant, indicating that Ser572 phosphorylation is also required for DLC2 dimerization ( Supplementary Fig. S2e ). Thus, this study demonstrates for the first time an interaction between members of the DLC family; DLC1 interacted with DLC2 in cells, yet the association was not influenced by PKA phosphorylation ( Supplementary Fig. S2f ), and DLC2 interacted with the DLC1 S549A and S549D mutants with similar affinity. 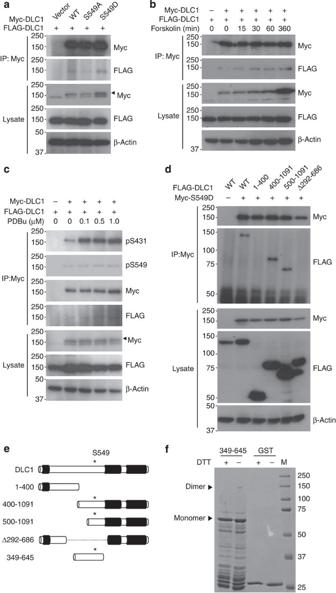Figure 5: Ser549 phosphorylation induces dimerization of DLC1. (a) DLC1 dimerizes with DLC1 and the S549D mutant but fails to interact with the S549A mutant. FLAG-DLC1 was coexpressed with Myc-DLC1, -S549A and -S549D in cells. Myc-DLC1 was immunoprecipitated with an anti-Myc antibody and immunoblotted with an anti-FLAG antibody. (b) Forskolin treatment induces the dimerization of DLC1. Myc- and FLAG-DLC1 were expressed in cells treated with forskolin for increasing durations. Myc-DLC1 was immunoprecipitated with an anti-Myc antibody and immunoblotted with an anti-FLAG antibody. (c) A phorbol ester induces the phosphorylation of Ser431 and slightly promotes the dimerization of DLC1. Myc- and FLAG-DLC1 were expressed in cells treated with increasing doses of PDBu. Total cell lysates were subjected to immunoprecipitation with an anti-Myc antibody followed by immunodetection using an anti-FLAG antibody. (d) DLC1 interacts via amino acids 500–686. The Myc-S549D mutant was tested for its interaction with various truncated Myc-DLC1 mutants by co-immunoprecipitation. (e) Schematic representation of the DLC1 deletion mutants used for mapping the interacting region. (f) DLC1 dimerizes via amino acids 349–645.In vitrokinase assay showing purified GST-DLC1 349-645 incubated with GST-PKA-Cα in the presence of ATP. The size of DLC1 was compared in sample buffer with or with dithiothreitol (DTT)-reducing agent. The DLC1 dimer and monomer are indicated. Figure 5: Ser549 phosphorylation induces dimerization of DLC1. ( a ) DLC1 dimerizes with DLC1 and the S549D mutant but fails to interact with the S549A mutant. FLAG-DLC1 was coexpressed with Myc-DLC1, -S549A and -S549D in cells. Myc-DLC1 was immunoprecipitated with an anti-Myc antibody and immunoblotted with an anti-FLAG antibody. ( b ) Forskolin treatment induces the dimerization of DLC1. Myc- and FLAG-DLC1 were expressed in cells treated with forskolin for increasing durations. Myc-DLC1 was immunoprecipitated with an anti-Myc antibody and immunoblotted with an anti-FLAG antibody. ( c ) A phorbol ester induces the phosphorylation of Ser431 and slightly promotes the dimerization of DLC1. Myc- and FLAG-DLC1 were expressed in cells treated with increasing doses of PDBu. Total cell lysates were subjected to immunoprecipitation with an anti-Myc antibody followed by immunodetection using an anti-FLAG antibody. ( d ) DLC1 interacts via amino acids 500–686. The Myc-S549D mutant was tested for its interaction with various truncated Myc-DLC1 mutants by co-immunoprecipitation. ( e ) Schematic representation of the DLC1 deletion mutants used for mapping the interacting region. ( f ) DLC1 dimerizes via amino acids 349–645. In vitro kinase assay showing purified GST-DLC1 349-645 incubated with GST-PKA-Cα in the presence of ATP. The size of DLC1 was compared in sample buffer with or with dithiothreitol (DTT)-reducing agent. The DLC1 dimer and monomer are indicated. Full size image Dimerization of DLC1 enhances the biological activities of DLC1 Next, we employed an inducible dimerization system, where DLC1 forms homodimers in the presence of small molecular B/B homodimerizer, to examine the functionality of dimerized DLC1. The FKBP-DLC1 fusion construct was created such that the FKBP V36-binding domain was inserted into DLC1, replacing Ser549 ( Fig. 6a ), and the interaction between Myc-FKBP-DLC1 and FLAG-FKBP-DLC1 in the presence of the homodimerizer was confirmed ( Fig. 6b ). To determine whether the induced dimerization of DLC1 could rescue the growth inhibitory effects of DLC1 containing a Ser549 deletion, the activities of FKBP-DLC1 were studied and compared in cells treated with or without the homodimerizer. FKBP-DLC1 was stably expressed in the mouse hepatoma cells ( Fig. 6c ), and in the presence of homodimerizer, these cells displayed a reduced growth rate, migratory potential and invasiveness ( Fig. 6d–f ). To confirm the role of dimerization in the growth suppression activity of DLC1 in vivo , the growth of subcutaneous tumours derived from FKBP-DLC1-expressing hepatoma cells treated with or without an intratumoural injection of homodimerizer was analysed. The development of tumours receiving a homodimerizer injection was delayed as compared with tumours injected with control buffer ( Fig. 6g ), and the size of homodimerizer-treated tumours was profoundly smaller than tumours in the control group ( Fig. 6h ). Taken together, these data suggest that the induced dimerization of DLC1 resulted in a more potent growth inhibitory activity. 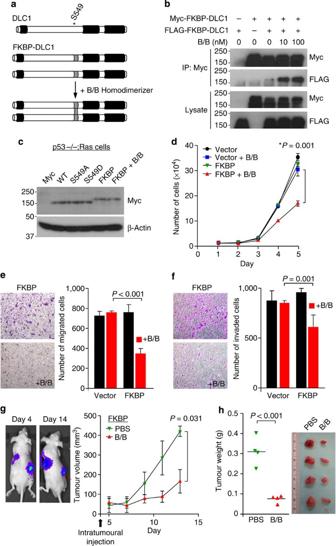Figure 6: Induced dimerization rescues the growth inhibitory activity of phosphorylation-deficient DLC1. (a) The inducible dimerization system demonstrates that the fusion of FKBP-DLC1 self-associates in the presence of B/B homodimerizer. FKBP inserted into DLC1 disrupts Ser549. (b) Myc- and FLAG-FKBP-DLC1 were expressed in HEK293 cells treated with increasing doses of homodimerizer. Addition of homodimerizer enhances the interaction between Myc- and FLAG-FKBP-DLC1. (c) Stable expression of FKBP-DLC1 in mouse hepatoma cells. (d) Growth curves of FKBP-DLC1 cells and vector control cells with or without homodimerizer treatment (n=3 for each group). (e) Transwell assay (n=3 for each group) showing that FKBP-DLC1 cells display a lower migratory potential when treated with homodimerizer. (f) An invasion assay (n=3 for each group) showing that the invasiveness of FKBP-DLC1 cells is reduced following homodimerizer treatment. (g) Intratumoural injection of homodimerizer in established subcutaneous xenografts (n=4 for each group). Tumour development is delayed in tumours injected with homodimerizer as compared with tumours injected with PBS. Images illustrating the luciferase signal in mice with subcutaneous injections of FKBP-DLC1 cells on day 4 and 14. Intratumoural injection of homodimerizer or PBS was initiated on day 4. (h) Tumours were excised and weighed at the end of the experiments. Error bar represents s.d. The results are expressed as the mean±s.d. Figure 6: Induced dimerization rescues the growth inhibitory activity of phosphorylation-deficient DLC1. ( a ) The inducible dimerization system demonstrates that the fusion of FKBP-DLC1 self-associates in the presence of B/B homodimerizer. FKBP inserted into DLC1 disrupts Ser549. ( b ) Myc- and FLAG-FKBP-DLC1 were expressed in HEK293 cells treated with increasing doses of homodimerizer. Addition of homodimerizer enhances the interaction between Myc- and FLAG-FKBP-DLC1. ( c ) Stable expression of FKBP-DLC1 in mouse hepatoma cells. ( d ) Growth curves of FKBP-DLC1 cells and vector control cells with or without homodimerizer treatment ( n =3 for each group). ( e ) Transwell assay ( n =3 for each group) showing that FKBP-DLC1 cells display a lower migratory potential when treated with homodimerizer. ( f ) An invasion assay ( n =3 for each group) showing that the invasiveness of FKBP-DLC1 cells is reduced following homodimerizer treatment. ( g ) Intratumoural injection of homodimerizer in established subcutaneous xenografts ( n =4 for each group). Tumour development is delayed in tumours injected with homodimerizer as compared with tumours injected with PBS. Images illustrating the luciferase signal in mice with subcutaneous injections of FKBP-DLC1 cells on day 4 and 14. Intratumoural injection of homodimerizer or PBS was initiated on day 4. ( h ) Tumours were excised and weighed at the end of the experiments. Error bar represents s.d. The results are expressed as the mean±s.d. Full size image Ser549 phosphorylation enhances DLC1 GAP activity against RhoA DLC1 is a RhoGAP that localizes to focal adhesions specific for RhoA and Cdc42 [9] , [27] , and the GAP activity of DLC1 contributes to its function. In agreement with reported studies, our data indicated that DLC1 significantly suppressed the activation of RhoA and Cdc42, but not Rac1, in stable hepatoma clones of DLC1 ( Fig. 7a ). Furthermore, Ser549 phosphorylation enhanced DLC1 GAP activity against active RhoA but not Cdc42, and the stable S549D clone had a reduced level of active RhoA as compared with the stable clone of DLC1 ( Fig. 7a , left panel). The impact of DLC1 dimerization on its RhoGAP activity was then explored. Hepatoma cells stably expressing FKBP-DLC1 were analysed for the level of active RhoA and Cdc42 ( Fig. 7b ). Following the addition of homodimerizer, the level of active RhoA was significantly reduced in cells expressing FKBP-DLC1 but not in the control cells, and the level of active Cdc42 remained unchanged. Together, our findings reveal that dimerization enhances the RhoGAP activity of DLC1, which contributes to the suppression of RhoA activity as well as the growth and migratory potential of cancer cells. To demonstrate that RhoA activity in cells is regulated by activated PKA via the phosphorylation of DLC1, RhoA activity was determined and compared between control cells (sh-control) and DLC1 knockdown cells (sh-DLC1) ( Fig. 7c ). Forskolin treatment significantly reduced RhoA activity in control cells, whereas the reduction of RhoA activity in DLC knockdown cells was insignificant. This result suggests that reduction of RhoA activity following forskolin treatment is partly mediated by DLC1. 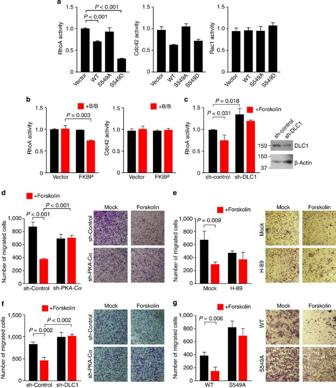Figure 7: Activated PKA signalling induces DLC1 Ser549 phosphorylation and enhanced RhoGAP activity. (a) GAP activity against RhoA is enhanced in S549D cells. Stable clones of DLC1, S549A, S549D and a vector control were subjected to small GTPase activation assays. Levels of active RhoA, Cdc42 and Rac1 were determined (n=3 for each group). (b) Stable clones of FKBP-DLC1 and a vector control were subjected to small GTPase activation assays. Levels of active RhoA and Cdc42 were determined in cells treated with or without homodimerizer treatment (n=3 for each group). The level of active RhoA is significantly reduced in FKBP-DLC1 cells treated with homodimerizer. (c) Forskolin reduces RhoA activity in a DLC1-dependent manner. RhoA activity was determined in sh-control cells and sh-DLC1 knockdown cells with and without forskolin treatment. Western blot analysis revealed the knockdown efficiency of DLC1. (d,e) Forskolin stimulation reduces the migration of SK-Hep-1 cells via activation of PKA. Cell migration was assessed using a Transwell assay, and the control cells, PKA-Cα knockdown cells and Sk-Hep-1 cells treated with and without H-89 were compared. (f) The effect of forskolin on the reduction of cell migration is lost in SK-Hep-1 DLC1 knockdown cells. (g) Inhibition of cell migration by forskolin treatment is mediated by the phosphorylation of DLC1 at Ser549. Stable DLC1 and S549A-expressing cells were assessed for the migration potential following forskolin treatment. Migration was suppressed in DLC1 cells, whereas there was no inhibition of migration in S549A cells following forskolin stimulation. Error bar represents s.d. The results are expressed as the mean±s.d. Figure 7: Activated PKA signalling induces DLC1 Ser549 phosphorylation and enhanced RhoGAP activity. ( a ) GAP activity against RhoA is enhanced in S549D cells. Stable clones of DLC1, S549A, S549D and a vector control were subjected to small GTPase activation assays. Levels of active RhoA, Cdc42 and Rac1 were determined ( n =3 for each group). ( b ) Stable clones of FKBP-DLC1 and a vector control were subjected to small GTPase activation assays. Levels of active RhoA and Cdc42 were determined in cells treated with or without homodimerizer treatment ( n =3 for each group). The level of active RhoA is significantly reduced in FKBP-DLC1 cells treated with homodimerizer. ( c ) Forskolin reduces RhoA activity in a DLC1-dependent manner. RhoA activity was determined in sh-control cells and sh-DLC1 knockdown cells with and without forskolin treatment. Western blot analysis revealed the knockdown efficiency of DLC1. ( d,e ) Forskolin stimulation reduces the migration of SK-Hep-1 cells via activation of PKA. Cell migration was assessed using a Transwell assay, and the control cells, PKA-Cα knockdown cells and Sk-Hep-1 cells treated with and without H-89 were compared. ( f ) The effect of forskolin on the reduction of cell migration is lost in SK-Hep-1 DLC1 knockdown cells. ( g ) Inhibition of cell migration by forskolin treatment is mediated by the phosphorylation of DLC1 at Ser549. Stable DLC1 and S549A-expressing cells were assessed for the migration potential following forskolin treatment. Migration was suppressed in DLC1 cells, whereas there was no inhibition of migration in S549A cells following forskolin stimulation. Error bar represents s.d. The results are expressed as the mean±s.d. Full size image As RhoA has an important role in actin cytoskeletal remodelling, we studied the effects of DLC1 Ser549 phosphorylation on the cytoskeletal architecture of SMMC7721 cells ( Supplementary Fig. S7a ). Upon transient transfection, DLC1 and the S549D mutant robustly inhibited serum-induced stress fibre formation, whereas the S549A mutant did not affect the stress fibre integrity. Staining of stable clone cells with a Golgi marker also demonstrated that the S549D mutant retarded the directional movement of the Golgi towards the edge of the wound ( Supplementary Fig. S7b ). These data agree with the notion that phosphorylation of DLC1 at Ser549 activates the GAP activity of DLC1 against RhoA and mediates the organization of the actin cytoskeleton. To further examine whether the functional effect of activated PKA signalling is due to the phosphorylation of DLC1, the migration of SK-Hep-1 PKA-Cα knockdown cells and SK-Hep-1 parental cells was examined in the presence and absence of a PKA inhibitor. Forskolin treatment efficiently reduced the migration of control cells, whereas both PKA-Cα knockdown cells and cells treated with H-89 were unresponsive to forskolin stimulation ( Fig. 7d ). Finally, these results further demonstrated that inhibition of cell migration by forskolin was abolished in DLC1 knockdown cells, suggesting that the inhibitory effect of PKA activation is mediated by DLC1 ( Fig. 7f ). As compared with the effect of forskolin stimulation on DLC1 and S549A stable clones, the inhibition induced by forskolin was lost in S549A-expressing cells but remained significant in WT DLC1 cells. Taken together, these data provide clear evidence for the role of activated PKA signalling in inducing the phosphorylation of DLC1 at Ser549 and therefore its dimerization and GAP activity against RhoA. Rho GTPases are molecular regulators that have roles in a number of normal cellular processes. They cycle between an active GTP-bound state and an inactive GDP-bound state, and they are regulated by GAPs and guanine-nucleotide-exchange factors (GEFs). Overexpression and activation of Rho GTPases are, however, observed in various human tumours [28] . Activation of the Rho pathway has been experimentally evident as a result of the loss of the DLC1 tumour suppressor in a physiologically relevant animal model [8] . Because of its frequent underexpression and heterozygous deletion in a wide variety of human cancers [4] , [8] , DLC1 is regarded as a significant GAP in the cancer genome [11] . Thus, study of the regulation of DLC1 GAP activity will foster a deeper understanding of the impact of Rho pathways in human cancers. The post-translational modification of DLC1 has recently garnered much attention as the most important regulatory mechanism of DLC1 activity, and kinases such as Akt, PKC and PKD have been shown to phosphorylate DLC1 at different residues and regulate its biological activities via RhoGAP-dependent as well as RhoGAP-independent pathways [6] , [20] , [29] . In this study, we evaluated the regulation of DLC1 activity by the cAMP/PKA pathway and found that PKA phosphorylates DLC1 at Ser431 and Ser549, which results in the dimerization, enhanced RhoGAP and tumorigenesis and metastasis inhibitory activities of DLC1 ( Fig. 8 ). We found that Ser431 is robustly phosphorylated in the S549D mutant without forskolin stimulation, whereas Ser431 is not phosphorylated in the S549A mutant regardless of forskolin. These results indicate that Ser431 is phosphorylated after Ser549 is phosphorylated by PKA. Thus, dimerization of DLC1 and the functional effect exerted by the S549D mutant could have resulted from dual phosphorylation at both Ser431 and Ser549. In accordance with the study of Scholz et al ., our data showed that a phorbol ester can induce DLC1 Ser431 but not Ser549 phosphorylation. This may explain why only minor DLC1 dimerization was induced by the addition of a phorbol ester [20] . Moreover, the phorbol ester induced the phosphorylation of DLC1 at Ser327 and Ser431, leading to its association with the 14-3-3 protein. Binding to the 14-3-3 protein may also mask the dimerization region of DLC1, which could have led to the weak interaction observed following phorbol ester treatment. 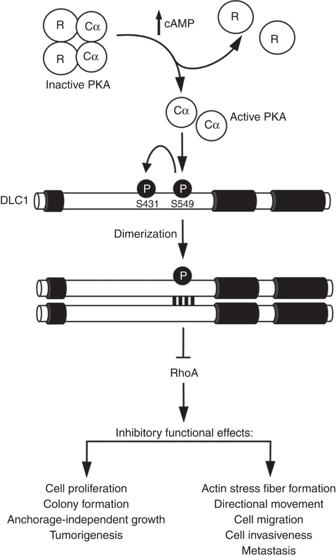Figure 8: A model for DLC1-positive regulation by PKA signalling. Active PKA phosphorylates DLC1 at Ser431 and Ser549, and Ser431 phosphorylation is dependent on the phosphorylation of Ser549. Phosphorylation of DLC1 at Ser549 mediates the dimerization of DLC1, leading to enhanced GAP activity against RhoA. Enhanced GAP activity leads to an increased inhibitory capacity of DLC1 in tumorigenesis and metastasis. Figure 8: A model for DLC1-positive regulation by PKA signalling. Active PKA phosphorylates DLC1 at Ser431 and Ser549, and Ser431 phosphorylation is dependent on the phosphorylation of Ser549. Phosphorylation of DLC1 at Ser549 mediates the dimerization of DLC1, leading to enhanced GAP activity against RhoA. Enhanced GAP activity leads to an increased inhibitory capacity of DLC1 in tumorigenesis and metastasis. Full size image In addition to DLC1, DLC2 has also been shown to dimerize via the unstructured region comprising residues 120–672 ( [30] ); however, the functional significance of DLC2 dimerization remains unclear. Our study provides the first demonstration of an interaction between DLC1 and DLC2, although this interaction is not affected by DLC1 Ser549 phosphorylation. DLC1 and DLC2 share similar structural organization, RhoGAP activity, focal adhesion localization and functional properties [31] , and although functional and molecular investigations of each member have been extensively reported in independent studies, functional data regarding the interplay between DLC1 and DLC2 are lacking. However, our demonstration of the interaction between DLC1 and DLC2 provides a strong rationale to further investigate the coupled signalling mechanisms that orchestrate the inhibition of tumour growth metastasis in human cancers. Using an inducible dimerization system, we further demonstrated the dependence of DLC1 dimerization for mediating its RhoGAP and growth suppression activities. Thus, the current study provides new knowledge regarding the fundamental regulation of DLC1 RhoGAP activity via structural dimerization. Apart from DLC1, other GAPs are regulated by dimerization; for example, the C-terminus of Slit-Robo GTPase-activating protein 2 (srGAP2) has been shown to be methylated by protein arginine methyltransferase 5, leading to the homodimerization of srGAP2 (ref. 32 ). The formation of srGAP2 homodimers promotes neuronal cell membrane protrusion and cell spreading. Semaphorin stimulates the RapGAP activity of plexin receptors in cells [33] , and the RapGAP activity of the purified plexin cytoplasmic region is stimulated by dimerization. Furthermore, the GAP activities of both srGAP2 and plexins are autoinhibited and activated by induced dimerization, implicating a GAP activation mechanism that is regulated by intermolecular interactions. Indeed, the RhoGAP activity of DLC1 has been shown to be inhibited by an intramolecular interaction with its SAM domain [34] , and association between the DLC1 SAM domain and tensin3 releases an autoinhibitory interaction in DLC1, thereby increasing its RhoGAP activity. Our data show that phosphorylation of DLC1 at Ser549 contributes to the association between DLC1 and tensin2 ( Supplementary Fig. S6 ). The DLC1 interaction with tensin2 is important for focal adhesion localization where it exerts its RhoGAP activity [24] , [26] . Thus, PKA may also contribute to DLC1 activity by regulating its interaction with tensin2 at focal adhesions. Here, we report that dimerization of DLC1 represents an activation mechanism for DLC1. This newly defined activation mechanism is regulated by PKA signalling, which is stimulated by an increase in the intracellular level of cyclic AMP (cAMP). The cAMP/PKA pathway has a profound role in the regulation of cell motility and cytoskeletal reorganization [35] . Furthermore, PKA has been shown to hinder multiple components of Rho signalling, which are crucial to cytoskeletal dynamics and cell movement [36] , [37] . PKA directly phosphorylates RhoA at Ser188 and inhibits its function by enhancing the interaction between RhoA and the Rho guanine-dissociation inhibitor [38] . In addition, PKA also negatively regulates the upstream activator of RhoA, and activated PKA associates and phosphorylates AKAP-Lbc at Ser1656. Phosphorylation of AKAP-Lbc subsequently recruits the binding of 14-3-3 dimers, which inhibits its Rho-GEF activity, thereby reducing the RhoA activity in cells [39] . Here, we reveal a signalling linkage between PKA and DLC1, two important molecular players involved in actin cytoskeletal reorganization. PKA mediates various physiological responses initiated by hormones. However, it remains unclear how the cAMP/PKA pathway regulates DLC1 in normal and cancerous cells, and the effect of the cAMP/PKA pathway on cell growth and motility is controversial, although activated cAMP/PKA signalling is clinically relevant in ovarian cancer [40] . Induction of cAMP stimulates the phosphorylation and nuclear translocation of cAMP response element-binding protein (CREB), and elevated expression levels of nuclear CREB have been observed in ovarian tumours as compared with normal ovarian tissues. Total CREB and phospho-CREB levels are also elevated in an ovarian cancer cell line as compared with a normal ovarian epithelial cell line. Additionally, the regulatory subunits of PKA are elevated in tumours and cancer cells and are associated with increased cell proliferation [41] , [42] . Conversely, the intracellular level of cAMP is suppressed by α6β4 integrin via the upregulation of cAMP phosphodiesterase during the migration of invasive breast carcinoma cells [43] . In HCC cell lines, cAMP exerts anti-proliferative effect via downregulation of cyclin A expression and inactivation of Akt [44] , [45] . Accordingly, we found that addition of forskolin reduced the migration and invasiveness of HCC cells ( Fig. 7 ). Others have reported that cAMP inhibits the mammalian target of rapamycin complex-1 and -2 activation via a PKA-dependent mechanism [46] . In a mouse model of inherited tumour syndrome Carney complex (CNC) with defect in the regulatory subunit 1α of PKA, there is evidence that prkar1a+/− (regulatory subunit 1α of PKA) mice developed HCC, while the PKA activity in these mice remained unchanged [47] . However, in another study, CNC patients with prkar1a mutations have been shown to develop a spectrum of carcinomas but not HCC [48] . These reported studies reveal an opposing role of cAMP/PKA pathway in different cellular contexts. DLC is frequently deleted in various human cancers. Cells with or without the presence of DLC1 might respond differentially to activated PKA pathway. The physiological relevance of PKA phosphorylation of DLC1 in HCC will be unveiled by the study and correlation of phosphorylation states of DLC1 and activity of PKA in HCC tissues. Cumulatively, the results of our current study advance the understanding of the regulatory mechanisms of DLC1. Our findings identify DLC1 as a novel substrate of the activated cAMP/PKA pathway and delineate how PKA regulates the RhoGAP and tumour suppression activities of DLC1 by structural dimerization. This new regulatory mechanism for DLC1, which has a prominent role in a broad range of human cancers, could have therapeutic implications. As aberrant activation of the Rho signalling pathway is implicated in the pathogenesis of human cancers, the modulation of GTPase regulators, such as GAPs and GEFs, may prevail over the direct inhibition of GTPases as an approach to combat the deregulated Rho pathway in human cancers. Constructs and reagents Expression constructs of Myc-tagged WT DLC1, the internal deletion mutant (Δ292-646), the RhoGAP mutant (K714E) and the GFP- and FLAG-tagged DLC2 were constructed as previously described [24] , [26] . DLC1 phospho-defective mutants (S431A, S549A and S341AS549A), phosphomimetic mutants (S431D and S549D) and the DLC2 S572A and S572D mutants were generated by PCR-based site-directed mutagenesis and verified by sequencing. The primers used for cloning are listed in Supplementary Table 1 . Amplified fragments were subcloned into pCS2+MT, FLAG-pcDNA3.1(+) (Invitrogen, Carlsbad, CA) and MSCV-PGK-PIG, which harbours a 6 × Myc tag at the N terminus (kindly provided by Professor Scott Lowe, Cold Spring Harbor). The PKA-Cα construct was a gift from Dr DY Jin (Department of Biochemistry, The University of Hong Kong). An oligomerization-inducible DLC1 was made by inserting the FKBP V36-binding domain into DLC1, such that it disrupts Ser549. The FKBP V36 domain is 327 bp in size. The Ser549 was first converted to Ile549 with the creation of an EcoRV site. The FKBP V36 fragment was inserted into DLC1 at the EcoRV site. The FKBP-DLC1 fusion fragment was then subcloned into the MSCV-PGK-PIG vector. The Myc- and FLAG-tagged FKBP-DLC1 constructs containing the deleted Ser549 residue were constructed in the pCS2+MT and pcDNA3.1+ vectors, respectively. Monoclonal anti-β-actin, anti-FLAG and anti-vinculin antibodies were purchased from Sigma-Aldrich (St Louis, MO). Antibodies against total CREB, pCREB (Ser133), PKA-Cα and phospho-PKA substrate (pPKAS) were obtained from Cell Signaling Technology (Danvers, MA). The anti-Myc and anti-DLC1 antibodies were purchased from Santa Cruz Biotechnology (Santa Cruz, CA) and BD Biosciences (San Jose, CA), respectively. Specific phospho-antibodies against pDLC1(Ser431) and pDLC1(Ser549) were custom made by Applied Biological Materials Incorporation (Richmond, BC, Canada). Forskolin, H-89 and PDBu were obtained from Calbiochem (San Diego, CA). B/B homodimerizer (AP20187) was purchased from Clontech (Mountain View, CA). Cell culture and retroviral transduction HEK293T cells, a human embryonic kidney cell line, and the HLE HCC cell line were purchased from the American Type Culture Collection, and the human HCC cell line SMMC7721 was obtained from the Shanghai Institute of Cell Biology. Mouse p53−/−;RasV12 hepatoblasts were provided by Professor Scott Lowe [8] . The establishment of DLC1 stable clones in mouse hepatoblasts was performed as previously described [6] . Phosphorylation of DLC1 was induced by treatment with 10 μM forskolin for 15 min before protein extraction. Inhibition of phosphorylation was conducted by pre-treating cells with 10 μM of H-89 for 1 h before forskolin stimulation. Soft agar assay A cell suspension (0.5 × 10 4 cells per 60-mm culture plate) was prepared in 0.4% agarose containing 2 × Dulbecco’s Modified Eagle's medium (DMEM) with high glucose and 20% fetal bovine serum and overlaid on a layer of 1% agarose containing the same medium. The cells were grown at 37 °C for 4 weeks to promote colony formation. At the end of the incubation, the number of colonies was counted. The data represent the mean of triplicate experiments, and the s.d. was also calculated. Flow cytometry Mouse hepatoma stable clones of DLC1 and its mutants were harvested, fixed with 0.5% paraformaldehyde in PBS and permeabilized with ice-cold 70% ethanol in PBS. The cells were then treated with 50 μg ml −1 RNaseA and stained with 50 μg ml −1 propidium iodide. The DNA contents of cell populations were determined using a FACSCalibur flow cytometer (BD Biosciences), and the results were analysed with WINMDI version 2.9. Apoptotic cells were defined as cells residing in the sub-G1 population. The percentage of cells in the sub-G1 phase for each stable clone was determined. The data represent the mean of triplicate experiments, and the s.d. was also calculated. Cell migration and invasion assays Mouse hepatoma cells (2 × 10 4 per well) were seeded into a Transwell plate (Corning, NY) for the migration assay, and 5 × 10 4 cells were plated in each well of a BD BioCoatMatrigel Invasion Chamber (BD Biosciences, Bedford, MA) for the invasion assay according to manufacturers’ instructions. Cells were suspended in serum-free medium in the upper chamber, and conditioned medium was added to the lower chamber. After 16 h of incubation, migrated or invaded cells were fixed and stained. Different fields of cells were photographed, and numbers of cells were counted. All of the experiments were performed in triplicate. Golgi orientation assay Cells were seeded onto coverslips and allowed to grow to confluence, and then a wound was made. At 5 h after the wound was made, the cells were fixed with 4% formaldehyde in PBS. The Golgi apparatus and nucleus were stained with GM130 (Sigma) and 4′,6-diamidino-2-phenylindole (DAPI) (Calbiochem), respectively. Golgi orientation was determined in cells along the leading edge of the wound. Cells in which the Golgi apparatus was within the sector facing the wound were scored as positive. Images were captured with a Leica Q550CW fluorescence microscope (Leica, Wetzler, Germany). A total of 300 cells were counted for each stable clone. All experiments were performed in triplicate. Subcutaneous injection and orthotopic liver implantation Mouse hepatoma stable clones of DLC1, S549A, S549D or FKBP-DLC1 cells were studied following injection into nude mice. For each stable clone, 1 × 10 5 cells were inoculated into the right flank of a 5-week-old male BALB/c nude mice. Tumour size was monitored for 14 days and estimated according to the following formula: volume=1/2 (largest diameter) × (smallest diameter) 2 . Tumours derived from DLC1, S549A and S549D cells were resected 2 weeks after subcutaneous injection for orthotopic liver implantation. All animals were killed and examined 3 weeks after implantation. The in vivo tumour formation was determined by bioluminescence (IVIS 100 Imaging System, Xenogen). For the intratumoural injection of homodimerizer into tumours derived from FKBP-DLC1 cells, the homodimerizer was injected 4 days after the subcutaneous injection of FKBP-DLC1 cells. A volume of 50 μl of 100 nM B/B homodimerizer was injected into the tumour on the right side of the animal every 2 days. The experiment was terminated after 2 weeks. The diameter of each tumour formed in the liver served as a measure of tumour size. Livers and lungs were excised and fixed for paraffin embedding. Paraffin sections were prepared and stained with hematoxylin-eosin (H&E) for histological examination. Tumours were analysed histologically for the presence of any aggressive features, such as an invasive tumour front and venous invasion. Lungs were analysed macroscopically or microscopically for any established metastasis. The animal work was conducted as previously described [6] . The experiments were performed according to the Animals (Control of Experiments) Ordinance (Hong Kong) and followed the University’s guidelines on animal experimentation. The experimental procedures for animal work have been approved by the Committee on the Use of Live Animals in Teaching and Research (CULATR). Co-immunoprecipitation and immunoblotting Experimental procedures for protein extraction, co-immunoprecipitation and western blotting have been previously described in detail [26] . Epitope-tagged proteins were immunoprecipitated from total cell lysates using specific antibodies against the tagged epitope. Endogenous DLC1 protein was immunoprecipitated with an anti-DLC1 antibody. Immunoprecipitated proteins were subjected to western blotting. To detect phosphorylation of DLC1, anti-pPKAS (Cell Signaling Technology) and custom-made anti-pDLC1 S431 and anti-pDLC1 S549 antibodies were used. In vitro kinase assay The in vitro kinase assay was performed as previously described [6] . Briefly, recombinant GST-DLC1 protein was generated using a GST expression system. GST-DLC1 or immunoprecipitated Myc-DLC1 were incubated with 0.5 mM ATP with or without 10 ng of GST-PKA-Cα (Cell Signaling Technology). The phosphorylation was detected with anti-pPKAS (Cell Signaling Technology), anti-pDLC1 (S341) or anti-pDLC1 (S549) antibodies by western blot analysis. To test for the dimerization of DLC1, the size of DLC1 was compared in sample buffer with or without the dithiothreitol-reducing agent. Small GTPase activation assay Small GTPase activity was evaluated using the G-LISA Small G-Protein Activation Assay (Cytoskeleton, Inc, Denver, CO), according to the manufacturer’s instructions. In brief, 4 × 10 4 or 8 × 10 4 mouse hepatoma stable clones of vector control, DLC1 WT, S549A, S549D and FKBP-DLC1 cells were seeded onto a 60-mm plate. A day after seeding, the cells were starved for 16 or 24 h in DMEM medium supplemented with 0.5% or 1% FBS. The cells were then further starved for another 8 or 24 h in DMEM medium. Cdc42 was induced by 10 ng ml −1 TNF-α, while RhoA and Rac1 were stimulated by the addition of conditioned medium for 2 min. Stress fibre formation assay A day after DNA transfection, stress fibre formation was induced by serum induction for 1 h before the fixation of transfected cells and immunofluorescence staining. DLC1 was stained with an anti-Myc antibody (Santa Cruz Biotechnology) followed by a fluorescein isothiocyanate (FITC)-conjugated secondary antibody. The nucleus of the cells was counterstained with DAPI. The F-actin was visualized using tetramethylrhodamine B isothiocyanate (TRITC)-labelled phalloidin (Sigma). The coverslips were mounted, and the images were captured using a fluorescence microscope. Statistical analysis The Student’s t -test was performed in GraphPad Prism 5.02 to determine whether differences between the experimental groups and the control groups were significant. A P -value less than 0.05 was regarded as statistically significant. Means and ±s.d. for each group were calculated and are shown. How to cite this article: Ko, F.C.F. et al . PKA-induced dimerization of the RhoGAP DLC1 promotes its inhibition of tumorigenesis and metastasis. Nat. Commun. 4:1618 doi: 10.1038/ncomms2604 (2013).